Sequence-based protein stabilization in the absence of glycosylation Asparagine-linked N -glycosylation is a common modification of proteins that promotes productive protein folding and increases protein stability. Although N -glycosylation is important for glycoprotein folding, the precise sites of glycosylation are often not conserved between protein homologues. Here we show that, in Saccharomyces cerevisiae , proteins upregulated during sporulation under nutrient deprivation have few N -glycosylation sequons and in their place tend to contain clusters of like-charged amino-acid residues. Incorporation of such sequences complements loss of in vivo protein function in the absence of glycosylation. Targeted point mutation to create such sequence stretches at glycosylation sequons in model glycoproteins increases in vitro protein stability and activity. A dependence on glycosylation for protein stability or activity can therefore be rescued with a small number of local point mutations, providing evolutionary flexibility in the precise location of N -glycans, allowing protein expression under nutrient-limiting conditions, and improving recombinant protein production. The presence of N -glycans assists protein folding, increases protein solubility, reduces aggregation and limits proteolysis [1] , [2] , [3] , [4] , [5] , while their specific structures affect glycoprotein function in development, cancer, inflammation and infection [3] , [6] . In eukaryotes, N -glycans are added to selected asparagine residues in nascent polypeptides co- and post-translocationally in the lumen of the endoplasmic reticulum (ER) by oligosaccharyltransferase (OTase) [7] , [8] , [9] , [10] . N -glycosylation by OTase occurs before substrate protein folding, as only flexible polypeptide substrate can bind at its active site [11] . The presence of Ser or Thr at the +2 position markedly increases glycosylation efficiency of asparagines, due to specific interactions with the peptide-binding site of OTase [11] , and such sequences are termed glycosylation sequons (N-x-S/T; x≠P). Asparagines in secondary structural elements tend to be inefficiently glycosylated [12] , [13] , as their reduced flexibility lowers their affinity to the OTase active site [11] . N -glycosylation therefore often occurs between secondary structural elements of folded proteins [14] . This allows N -glycans to optimally assist productive protein folding by their hydrophilic bulk lowering the entropy of the protein unfolded state and acting as nucleation sites for local folding of nascent glycopolypeptide chains [2] . N -glycans can also increase protein stability by making direct contacts with amino acids in the folded protein [15] , [16] , increasing overall protein solubility [17] , shielding exposed hydrophobic surfaces [18] and limiting proteolysis [19] . In the ER, N -glycans act as signals to locally recruit ER chaperones to assist in glycoprotein oxidative folding and are important in glycoprotein quality control and degradation [2] , [20] , [21] , [22] . Although N -glycans are important for protein folding and function, the precise sites of glycosylation within a protein are not generally conserved in homologues. Here, we study the extent to which peculiar amino-acid sequences can functionally replace N -glycosylation sites. We show that clusters of like-charged amino acids in place of N -glycosylation sequons can impart local protein stability and improve protein function in the absence of glycosylation. Sequence analysis of yeast cell wall N -glycoproteins In the absence of a nitrogen source and in the presence of a nonfermentable carbon source, bakers’ yeast S. cerevisiae ceases vegetative growth and enters sporulation [23] . This results in large changes to many aspects of yeast biology including remodelling of the cell wall. Key enzymes involved in this process are the GAS family of glucanases/transglycosidases. Gas1p is a major cell-wall protein during vegetative growth while its functionally equivalent paralogue Gas2p is predominantly expressed during sporulation [24] , [25] . Gas1p and Gas2p share 45% sequence identity, conserved secondary structure and identical disulphide bond connectivity [26] , [27] . However, Gas1p has 10 N -glycosylation sequons while Gas2p has only 1. This prompted us to test if other sporulation-induced proteins also had few glycosylation sequons. This analysis showed that glycoproteins upregulated in sporulation did have fewer glycosylation sequons than their paralogues expressed during vegetative growth ( Fig. 1a ). The nutrient limitations that induce sporulation may provide a selective pressure for reducing flux through the energetically expensive N -glycosylation pathway, resulting in loss of N -glycosylation sequons from sporulation-specific proteins. 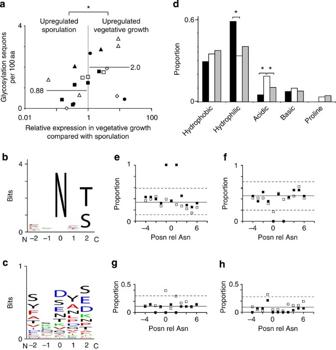Figure 1: Equivalent sequences to glycosylation sites in yeast cell-wall proteins. (a) Glycosylation sequon density is higher in glycoprotein paralogues upregulated in vegetative growth than in those upregulated in sporulation. Paralogues of black squares, Gas1p; white squares, Mkc7p; black circles, Exg1p; black triangles, Plb1p; white triangles, Ecm33p; and white diamonds, Crh1p. Horizontal bars show mean for each group. *P=0.01, 2-sided Mann–Whitney test. (b) Weblogo representation of aligned experimentally validated glycosylation sites and (c) corresponding sequences in homologues lacking glycosylation sites. (d) Proportion of hydrophilic, hydrophobic, acidic and basic amino acids in validated sites (black), corresponding sequences lacking sequons (white) and in the entire protein sequences of all homologues analysed (grey). *P<0.005, Fisher’s exact test. Position specific proportion of (e) hydrophilic, (f) hydrophobic, (g) acidic and (h) basic amino acids for validated glycosylation sites in yeast cell-wall proteins (black squares) and corresponding sequences in paralogues lacking sites (white squares). Horizontal lines indicate mean values of the entire protein sequence of all homologues analysed (full) and the values at whichP=0.001 by Fisher’s exact test compared with this mean for a given position (dashed). Figure 1: Equivalent sequences to glycosylation sites in yeast cell-wall proteins. ( a ) Glycosylation sequon density is higher in glycoprotein paralogues upregulated in vegetative growth than in those upregulated in sporulation. Paralogues of black squares, Gas1p; white squares, Mkc7p; black circles, Exg1p; black triangles, Plb1p; white triangles, Ecm33p; and white diamonds, Crh1p. Horizontal bars show mean for each group. * P =0.01, 2-sided Mann–Whitney test. ( b ) Weblogo representation of aligned experimentally validated glycosylation sites and ( c ) corresponding sequences in homologues lacking glycosylation sites. ( d ) Proportion of hydrophilic, hydrophobic, acidic and basic amino acids in validated sites (black), corresponding sequences lacking sequons (white) and in the entire protein sequences of all homologues analysed (grey). * P <0.005, Fisher’s exact test. Position specific proportion of ( e ) hydrophilic, ( f ) hydrophobic, ( g ) acidic and ( h ) basic amino acids for validated glycosylation sites in yeast cell-wall proteins (black squares) and corresponding sequences in paralogues lacking sites (white squares). Horizontal lines indicate mean values of the entire protein sequence of all homologues analysed (full) and the values at which P =0.001 by Fisher’s exact test compared with this mean for a given position (dashed). Full size image Given the importance of N -glycosylation for protein folding, we investigated if the equivalent positions of N -glycans in paralogues that lacked a sequon at that particular site had compensatory amino-acid sequences. For this, we used a set of experimentally validated yeast glycosylation sites [13] , [28] , [29] , [30] . Sequence analysis of positions in paralogues corresponding to these sites showed that they had more acidic amino acids compared with both validated glycosylation sites and the average amino-acid composition of the whole protein set ( Fig. 1b–d ). This enrichment was only significant in the immediate vicinity of the residues corresponding to the location of the glycosylation sequon ( Fig. 1e–h ), although the high sequence diversity in this analysis precluded the identification of more specific patterns. Functional complementation of glycosylation sites in yeast To test if these clusters of acidic amino acids served to provide local intrinsic stability to the protein even in the absence of N -glycosylation, we expressed and purified the model glycoproteins yeast Gas1p and Gas2p as secreted MBP fusions in E. coli and S. cerevisiae . Given Gas1p has many more N -glycosylation sequons than Gas2p, we predicted that Gas2p would be more stable than Gas1p when expressed without N -glycosylation in E. coli . Circular dichroism (CD) spectroscopy of E. coli -expressed protein was consistent with MBP-Gas2 containing more helical secondary structure than MBP-Gas1, while the native glycosylated forms of these S. cerevisiae -expressed proteins showed equivalent CD spectra ( Fig. 2a,b ). MS analysis of the disulphide bond connectivity by non-reducing tryptic peptide mapping showed that both E. coli -expressed MBP-Gas1 and MBP-Gas2 had incorrect connectivity compared with native protein expressed in yeast ( Supplementary Tables 1 and 2 ) [26] , [27] . To enable comparison with native glycosylated MBP-Gas1 and MBP-Gas2, we created disulphide shuffled forms of these S. cerevisiae -expressed proteins. CD spectra of these disulphide shuffled forms of MBP-Gas1 and MBP-Gas2 were similar to their native forms ( Fig. 2a,b ). This is consistent with the increased stability and secondary structure in nonglycosylated MBP-Gas2 compared with nonglycosylated MBP-Gas1 being local effects that influence secondary structure formation. That is, the absence of N -glycosylation at the 10 glycosylation sites in Gas1p strongly affected local formation of secondary structural elements, whereas this affect was not as strong in Gas2p, which with only a single glycosylation site does not natively rely on N -glycosylation for stability to the extent of Gas1p. 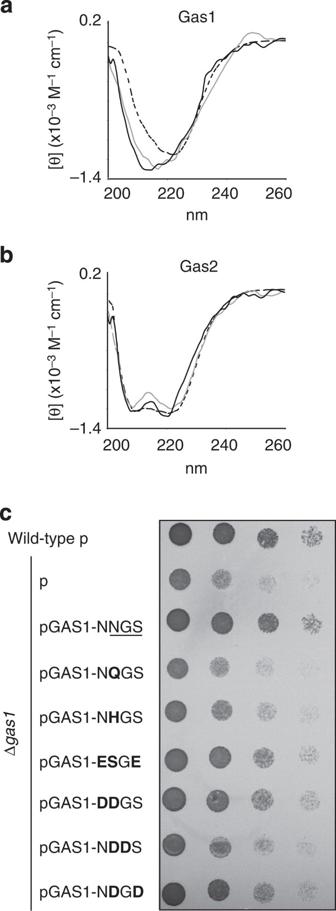Figure 2: Structure and function of Gas1p and Gas2p glycosylation site variants. (a) CD spectra of MBP-Gas1 and (b) MBP-Gas2 produced inE. coli(dashed black), orS. cerevisiaenative (solid black) or disulphide-shuffled (solid gray). Mean residue ellipticity is shown. (c) Growth of yeast with wild-type Gas1p (wild type, pGAS1-NNGS) and Asn40 glycosylation site variants. The native Asn40 sequon is underlined. Point mutations in variants are bold. Figure 2: Structure and function of Gas1p and Gas2p glycosylation site variants. ( a ) CD spectra of MBP-Gas1 and ( b ) MBP-Gas2 produced in E. coli (dashed black), or S. cerevisiae native (solid black) or disulphide-shuffled (solid gray). Mean residue ellipticity is shown. ( c ) Growth of yeast with wild-type Gas1p (wild type, pGAS1-NNGS) and Asn40 glycosylation site variants. The native Asn40 sequon is underlined. Point mutations in variants are bold. Full size image We next tested if the Gas2p sequences corresponding to Gas1p glycosylation sites were functionally equivalent in vivo . Yeast cells with deletion of GAS1 showed reduced growth compared with wild-type cells, which was complemented by overexpression of native Gas1p ( Fig. 2c ). Gas1p is glycosylated at Asn40 (NN 40 GS) [13] and expression of variant Gas1-N40Q lacking this glycosylation site did not complement loss of GAS1 ( Fig. 2c ). While Asn-Gln site-directed mutagenesis is routinely used to test the importance of particular glycosylation sites in glycoprotein folding and function, the conformational preferences of Gln are very different to those of Asn, while His is more similar to Asn [31] . Expression of variant Gas1-N40H only partially complemented loss of GAS1 ( Fig. 2c ). This lack of complementation indicated that glycosylation at Asn40 was required for Gas1p function in the context of the native sequence. However, replacing this stretch of Gas1p with the corresponding sequence from Gas2p ( 39 ESGE 42 ; Supplementary Fig. 1a ) restored growth, as did point mutation to insert proximal Asp residues ( Fig. 2c ), while retaining the conserved Gly41 ( Supplementary Fig. 1b ). The dependency of in vivo Gas1p function on glycosylation at Asn40 could therefore be rescued by a small number of compensatory point mutations introducing local clusters of negatively charged residues. Stabilization of unglycosylated human interferon-β Animal glycoproteins are not generally required to be expressed under such severe nutrient limitations as during yeast sporulation. However, human glycoproteins are often expressed for biotechnological purposes in bacteria that lack glycosylation systems. Such a protein is the human glycoprotein hormone interferon-β (IFNβ) [32] . The single N -glycosylation site in human IFNβ is not strictly conserved in orthologues and paralogues ( Fig. 3a , Supplementary Fig. 2 ), and in these proteins is often replaced by clusters of acidic amino acids similar to those observed in place of N -glycosylation sites in yeast proteins ( Fig. 1 , Supplementary Fig. 1 ). To test if such a sequence would increase IFNβ stability in the absence of glycosylation, we expressed and purified IFNβ as wild type and glycosylation site variant (Asn101Asp) forms from E. coli and refolded these proteins in vitro . Guanidinium-induced unfolding equilibria showed that at physiologically relevant pH 7.5 this point mutation increased stability (ΔΔ G 0 −9 kJ mol −1 , Fig. 3b ). In contrast, at pH 5.0 the ΔΔ G 0 was negligible ( Fig. 3c ). We propose that this is consistent with stabilization of the IFNβ N101D variant at pH 7.5 through reduced entropy of the unfolded state due to charge-charge repulsion between Asp101 and Glu102 favouring a local turn or extended structure similar to the structure of Asn101 and Glu102 in folded native IFNβ [18] , or stabilization of the native state [33] , [34] . At pH 5 there is a lower probability that both these residues will be simultaneously deprotonated (negatively charged) in a given protein molecule, consistent with the lack of stabilization in the IFNβ N101D variant. The overall higher stability for both protein forms at pH 5.0 than at pH 7.5 is likely due to increased distance from the predicted pI of IFNβ (~9.0). This confirmed that local clusters of negatively charged amino acids could increase protein stability in the absence of glycosylation in homologues of human IFNβ. To confirm that stable IFNβ N101D retained native activity, we performed a cell culture growth inhibition assay ( Fig. 3d ). Stable IFNβ N101D showed significantly higher specific activity than IFNβ wild type ( Fig. 3d ), correlating increased thermodynamic stability with improved protein function in this assay. This suggested that it is possible for IFN proteins to have either N -glycosylation sites or sequence stretches that can play a similar role in protein folding and stability. 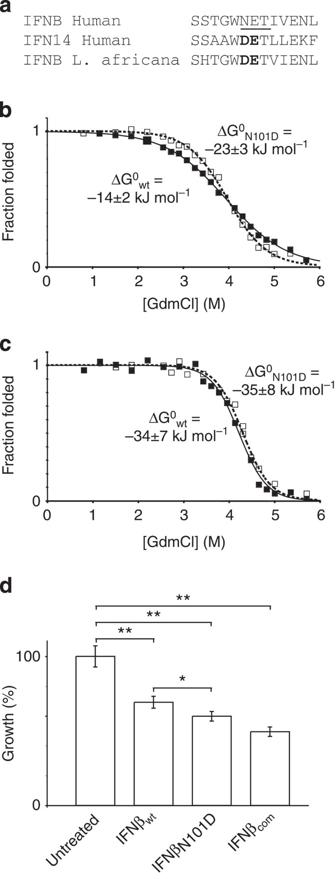Figure 3: Stability and activity of human IFNβ variants. (a) Alignment of human IFNβ and a selected orthologue and paralogue. The IFNβ glycosylation sequon is underlined and corresponding clusters of acidic amino acids are in bold. (b) Guanidinium induced equilibrium unfolding of IFNβ wild-type and IFNβN101Dvariant as measured by intrinsic tryptophan fluorescence and fitted to the two-state model of protein folding at pH 7.5 and at (c) pH 5.0. Solid line, IFNβ wild type; dashed line, IFNβN101D. (d) Activity of IFNβwt, IFNβN101Dand IFNβCom(Commercial nonglycosylated protein) in a cell culture growth inhibition assay. Values show mean of percent cell survival relative to untreated cells,n>8; Error bars show s.e.m.; *P=0.002, **P=10−7, student’st-test. Figure 3: Stability and activity of human IFNβ variants. ( a ) Alignment of human IFNβ and a selected orthologue and paralogue. The IFNβ glycosylation sequon is underlined and corresponding clusters of acidic amino acids are in bold. ( b ) Guanidinium induced equilibrium unfolding of IFNβ wild-type and IFNβ N101D variant as measured by intrinsic tryptophan fluorescence and fitted to the two-state model of protein folding at pH 7.5 and at ( c ) pH 5.0. Solid line, IFNβ wild type; dashed line, IFNβ N101D . ( d ) Activity of IFNβ wt , IFNβ N101D and IFNβ Com (Commercial nonglycosylated protein) in a cell culture growth inhibition assay. Values show mean of percent cell survival relative to untreated cells, n >8; Error bars show s.e.m. ; * P =0.002, ** P =10 −7 , student’s t -test. Full size image Stabilization at an inefficiently glycosylated sequon Asparagines in sequons generally show macroheterogeneity with not all of the protein pool glycosylated, and almost all sequons are modified to some extent [9] . We therefore tested whether essentially unmodified sequons could also be subject to sequence-based stabilization. For this purpose we studied the paralogous yeast proteins Ost3p and Ost6p, which are accessory subunits of OTase [7] , [13] . The ER lumenal domain of Ost3p has a single sequon at Asn33, which is not detectably glycosylated [35] ( Fig. 4a and Supplementary Fig. 3 ), while Ost6p has no sequons and contains a cluster of acidic amino acids at the position corresponding to the Ost3p sequon ( Supplementary Fig. 4 ). The ER lumenal domain of Ost6p is more easily expressed than that of Ost3p in E. coli [30] and shows activity in an in vitro peptide-binding assay when Ost3p does not [36] . To test if the higher in vitro activity of Ost6p relative to Ost3p correlated with increased thermodynamic stability of Ost6p, we performed guanidinium-induced equilibrium unfolding of Ost6 and Ost3 purified from E. coli . This showed that Ost6 (Δ G 0 =−79±10 kJ mol −1 ) was more stable than Ost3 (Δ G 0 =−28±5 kJ mol −1 ) ( Fig. 4b,f ), consistent with the presence of clusters of like-charged amino acids in place of an unused glycosylation sequon increasing thermodynamic stability and activity. To test this in the context of Ost6p, we introduced a glycosylation sequon in Ost6 at the equivalent position to the Ost3 sequon, and tested in vitro stability and peptide-binding activity. This variant of Ost6 with a glycosylation sequon had both reduced stability compared with wild-type Ost6 (Ost6 D38N ΔΔ G 0 =20 kJ mol −1 ) ( Fig. 4f,g ), and essentially eliminated in vitro peptide-binding activity ( Fig. 4l,m ). We next tested whether the stability and in vitro activity of Ost3 could be increased by targeted point mutation at the unused sequon in Ost3. We first introduced an acidic Asp in place of Asn33, which increased stability compared with wild-type protein (Ost3 N33D ΔΔ G 0 =−16 kJ mol −1 ) ( Fig. 4c ), but did not result in a detectable increase in in vitro peptide binding ( Fig. 4h,i ). However, Ost3p orthologues lack sequons at this position and instead typically possess clusters of basic amino acids, while Ost6p orthologues have acidic residues at this position ( Supplementary Fig. 4 ). This difference may depend on Ost3p- and Ost6-specific charge distributions on a neighbouring α-helix ( Supplementary Fig. 5 ). We therefore tested two additional variants with clusters of either acidic or basic like-charge. While Ost3 N33D,K34D ( 30 KLA DD SPKK 38 ) was less stable (ΔΔ G 0 =6 kJ mol −1 ) ( Fig. 4d ), Ost3 N33K ( 30 KLA K KSPKK 38 ) was more stable than Ost3 N33D and wild-type Ost3 (ΔΔ G 0 =−27 kJ mol −1 ) ( Fig. 4e ). Optimal stabilization was therefore achieved through minimal mutations providing a cluster of like-charged residues. This stable Ost3 N33K showed increased in vitro binding of several peptides ( Fig. 4j,k ). These peptides contained aromatic amino acids, complementary to Phe102 in the peptide-binding groove of Ost3, a key determinant of transient nascent polypeptide tethering by Ost3 crucial to its function in modulating OTase activity in vivo [30] , [36] . The additional thermodynamic stability of Ost3 N33K therefore enabled its function to be investigated in this in vitro assay. 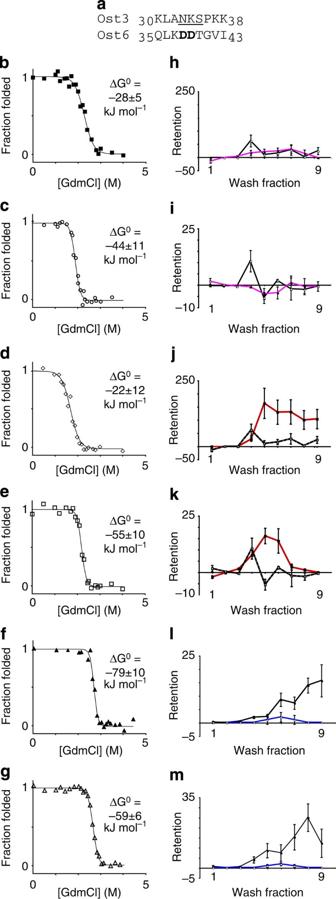Figure 4: Stability and function of yeast Ost3 and Ost6 variants. (a) Alignment of Ost3 and Ost6. The Ost3 glycosylation sequon is underlined and corresponding cluster of acidic amino acids in Ost6 are in bold. Guanidinium induced equilibrium unfolding of (b) Ost3, (c) Ost3N33D, (d) Ost3N33D, K34D, (e) Ost3N33K, (f) Ost6 and (g) Ost6D38N, as measured by intrinsic tryptophan fluorescence and fitted to the two-state model of protein folding. Peptide binding to Ost3 wild type (black) and Ost3N33D(purple) by peptides (h) LVIWINGDK (m/zof 1,057.6+) and (i) FFYSNNGSQFYIR (m/zof 1,642.8+), to Ost3 wild type (black) and Ost3N33K(red) by peptides (j) LVIWINGDK (m/zof 1,057.6+) and (k) FFYSNNGSQFYIR (m/zof 1,642.8+), and to Ost6 wild type (black)36and Ost6D38N(blue) by (l) LVIWINGDK (m/zof 1,057.6+) and (m) AGLTFLVDLIK (m/zof 1,189.7+). Values show mean of triplicates, error bars show s.e.m. Figure 4: Stability and function of yeast Ost3 and Ost6 variants. ( a ) Alignment of Ost3 and Ost6. The Ost3 glycosylation sequon is underlined and corresponding cluster of acidic amino acids in Ost6 are in bold. Guanidinium induced equilibrium unfolding of ( b ) Ost3, ( c ) Ost3 N33D , ( d ) Ost3 N33D, K34D , ( e ) Ost3 N33K , ( f ) Ost6 and ( g ) Ost6 D38N , as measured by intrinsic tryptophan fluorescence and fitted to the two-state model of protein folding. Peptide binding to Ost3 wild type (black) and Ost3 N33D (purple) by peptides ( h ) LVIWINGDK ( m/z of 1,057.6 + ) and ( i ) FFYSNNGSQFYIR ( m/z of 1,642.8 + ), to Ost3 wild type (black) and Ost3 N33K (red) by peptides ( j ) LVIWINGDK ( m/z of 1,057.6 + ) and ( k ) FFYSNNGSQFYIR ( m/z of 1,642.8 + ), and to Ost6 wild type (black) [36] and Ost6 D38N (blue) by ( l ) LVIWINGDK ( m/z of 1,057.6 + ) and ( m ) AGLTFLVDLIK ( m/z of 1,189.7 + ). Values show mean of triplicates, error bars show s.e.m. Full size image We show that targeted introduction of like-charged amino acids at N -glycosylation sequons is a generally applicable technique for increasing the stability of normally N -glycosylated proteins when expressed from more efficient expression systems such as E. coli . The targeted nature of this approach also limits any unanticipated affects on protein structure or function of non-targeted mutagenesis. The presence of a sequon rather than a compensatory sequence at a specific location in a given protein may also depend on its protein context. For example, experimental [1] , [16] and computational [37] characterization of variants of CD2 adhesion domain from human (which is glycosylated) and rat (which is not glycosylated) has shown that gain of glycosylation mutations in Rat CD2 do not immediately increase protein thermodynamic stability. However, acquisition of two additional mutations proximal to the newly glycosylated Asn introduces specific glycan–protein interactions, which lead to the formation of high-occupancy hydrogen bonds and stabilize the glycosylated protein. Alternatively, while loss of glycosylation mutations in human CD2 destabilizes the protein, two additional nearby mutations rescue stability and function [38] . Experimentally, Asn-Gln site-directed mutagenesis is commonly used as a proxy for loss of glycosylation at a given site. Such a mutation may show if glycosylation at that site is important for protein folding, stability or activity, in the context of an otherwise unchanged protein sequence. However, our bioinformatics, in vitro and in vivo results here show that such a requirement could in general be easily rescued by evolutionary acquisition of a small number of stabilizing point mutations. The exact reasons why particular glycoproteins have N -glycosylation sites at specific locations are undoubtedly complex, depending not only on their affect on global protein stability but also on evolutionary history and the many roles of N -glycans in influencing protein function. Sequence analyses Families of yeast glycoproteins with members expressed predominantly during vegetative growth or sporulation were identified from expression data [23] and UniProt BLAST with a cutoff of e-4. Sequence analysis was performed based on a set of experimentally validated occupied glycosylation sites in S. cerevisiae cell-wall glycoproteins (28 sites in 13 glycoproteins) [13] , [28] , [29] . Homologues to these from S. cerevisiae were identified with UniProt BLAST with a cutoff of e-4, and each of these sets of homologous proteins and glycoproteins were aligned with ClustalW. For each experimentally validated glycosylation site, aligned sequences of homologous proteins were identified that did not contain a glycosylation sequon at that position (41 sequences). The characteristics of the amino-acid sequences flanking these sites (glycosylation sites, and corresponding sequences in homologues lacking glycosylation sites) were determined through a non-gapped alignment visualized with WebLogo [39] and amino-acid composition (hydrophilic, hydrophobic, acidic or basic). pI of the amino-acid sequences was determined with ProtParam [40] . Cloning and mutagenesis DNA encoding the ER lumenal domain of S. cerevisiae Gas2p as predicted in the UniProt Knowledgebase (position 25 to 531 of Gas2p/Q06135/YLR343W) was cloned into the pMAL-p2x vector, using PCR primers incorporating Bam HI and Hin dIII restriction sites, to give pMAL-GAS2. DNA encoding the GAS1 genomic locus (GAS1/P22146/YMR307W including 1 kb up and downstream) was cloned into the pRS415 vector to give pRS415-GAS1. Blunt ended DNA encoding mature MBP-Gas1 or MBP-Gas2 was amplified using PCR primers incorporating a C-terminal His-tag, phosphorylated with T4 polynucleotide kinase, and ligated into blunt ended DNA amplified from pRS415-GAS1 excluding DNA encoding mature GAS1 (ref. 41) [41] . This produced pRS415-MBP-GAS1-His and pRS415-MBP-GAS2-His, which encoded MBP-Gas1-His or MBP-Gas2-His with the native Gas1p signal sequence under the control of the native GAS1 promoter and terminator. DNA encoding the mature protein sequence of IFNβ as predicted in the UniProt Knowledgebase (position 22 to 187 of P01574) with Cys17 changed to Ser [32] and with an N-terminal decaHis-tag, optimized for E. coli protein expression was synthesized and cloned into the pJexpress404 expression vector (DNA 2.0). DNA sequence encoding a C-terminal FLAG-tag was inserted in S. cerevisiae OST3 on plasmid YEp352 (ref. 42) [42] using site-directed mutagenesis [41] to create pOST3-FLAG. Point mutation of GAS1, IFNβ and OST3 were performed by site-directed mutagenesis [41] . Cell culture and protein purification BY4741 (MATa his3Δ1 leu2Δ0 met15Δ0 ura3Δ0 ) yeast cells and the Δgas1 mutant derivative thereof (Open Biosystems) was transformed with pRS415, pRS415-GAS1 or variants using standard protocols. Cells were diluted to equal densities at OD 600 nm , serially 10-fold diluted, equal volumes spotted to minimal media agar plates and incubated at 30 o C. TOP10 E. coli cells carrying the plasmids encoding IFNβ, Ost6 (pHis10-OST6L [43] ), Ost3 (pHis10-OST3L [43] ) or variants thereof were grown in LB media, and cells carrying pMAL-Gas1 (ref. 36) [36] or pMAL-Gas2 were grown in LB-glucose media. Media was supplemented with 100 mg l −1 ampicillin. Protein expression was induced by addition of IPTG to 1 mM at an OD 600 nm of 0.7. After incubation for 4 h at 37 °C the cells were collected by centrifugation. MBP-Gas1 and MBP-Gas2 were purified as previously described [36] , except that protein was eluted with 10 mM maltose. Yeast cells carrying pRS415-MBP-GAS1-His or pRS415-MBP-GAS2-His were grown in minimal media at 30 °C with shaking and collected at an OD 600 nm of 1.0. Cells were resuspended in 50 mM phosphate buffer pH 7.5, 150 mM NaCl, 1 × protease inhibitor cocktail (Roche) and 1 mM PMSF, and lysed by French Press. Proteins were purified using TALON resin (Clontech) and eluted in 50 mM phosphate buffer pH 7.5, 150 mM NaCl and 250 mM imidazole. The TALON resin eluate was then applied to amylose-agarose beads and purified as previously described [36] , except that protein was eluted with 10 mM maltose. Disulphide-shuffled protein was produced by reduction in 6 M guanidinium chloride, 50 mM phosphate buffer pH 7.5 with 10 mM DTT, buffer exchange into 1 M guanidinium chloride, 50 mM phosphate buffer pH 7.5 with 0.1 mM CuSO 4 and incubation at 25 °C for 2 h. Protein was then buffer exchanged into 20 mM phosphate buffer pH 7.5, 200 mM NaCl and 1 mM EDTA. Collected cells expressing IFNβ variants were resuspended in 50 mM phosphate buffer pH 7.5, 150 mM NaCl, 1 × protease inhibitor cocktail (Roche) and 1 mM PMSF, and lysed by French Press. Inclusion bodies were recovered by sequential centrifugation at 18,000 rcf. The pellets were washed with 1 ml 50 mM phosphate buffer pH 7.5 and 150 mM NaCl and re-centrifuged three times. The washed pellets containing inclusion bodies were resolublized in 6 M guanidinium chloride, 50 mM phosphate buffer pH 7.5 and 1 mM β-mercaptoethanol and incubated at 37 °C for 16 h. His-tagged IFNβ was purified using TALON resin (Clontech) and eluted in 6 M guanidinium chloride, 50 mM phosphate buffer pH 5.0 and 1 mM β-mercaptoethanol. The pH was adjusted to pH 7.5 with other constituents remaining constant, DTT was added to 20 mM and the protein was incubated at 37 °C for 1 h. Protein was buffer exchanged with PD-10 columns (GE Healthcare) into 50 mM phosphate buffer pH 7.5 and 6 M guanidinium chloride. Cysteines were oxidized to cystine by addition of 0.1 mM CuSO 4 and incubation at 25 °C for 2 h. Oxidation was quenched by addition of 1mM EDTA, and oxidized IFNβ was buffer exchanged with PD-10 columns into 50 mM phosphate buffer pH 7.5 and 25% glycerol at 4 °C. Cells expressing N-terminally His-tagged Ost6, Ost3 or variants thereof were resuspended in ice cold 50 mM Potassium Phosphate, pH 7.5, 150 mM NaCl, 10 mM Imidazole, 1 × complete mini EDTA free protease inhibitor (Roche) and 1 mM PMSF, and lysed by French Press. Protein was purified from clarified whole-cell extract using TALON resin and eluted with 200 mM imidazole. Proteins were buffer exchanged with PD-10 columns into 50 mM potassium phosphate buffer pH 7.0 and 1 mM EDTA. Yeast with pOST3 or pOST3-FLAG were grown in minimal media at 30 °C and collected at mid log phase. Proteins were denatured in SDS sample buffer, incubated for 1 h at 37 °C with 1 × G5 buffer in the presence or absence of Endo H [13] , separated by SDS-PAGE, transferred to nitrocellulose membrane and probed with an α-FLAG antibody. In vitro protein analysis CD spectra were obtained using a Jasco J-710 spectrometer (Jasco, Japan) as described [44] . Free energies of stabilization (Δ G 0 ) were determined based on the two-state model of protein folding [45] as described [30] . To determine the equilibrium transitions, intrinsic tryptophan fluorescence of proteins was measured in different concentrations of guanidinium chloride in 50 mM potassium phosphate pH 7.5 or 5.0, and 150 mM NaCl at 25 °C. Δ G 0 and cooperativity were determined from a non-linear least-squares 6 parameter fit to the data points [45] , with uncertainty estimates from the corresponding six-parameter fits. Ost3 and Ost6 peptide-binding affinity chromatography was performed as described [36] . Briefly, tryptic peptides from MBP-Gas1p were applied to peptide-affinity chromatography columns containing MBP-Ost3, MBP-Ost3 N33K , MBP-Ost6 or MBP-Ost6 D38N bound to amylose-agarose resin with or without pre-reduction with DTT. Peptides were eluted with physiological buffer, fractions collected, and peptides in the load and elution fractions were detected with MALDI-TOF-MS. Peptide retention was determined by the relative abundance of each peptide in wash fractions compared with the load, in oxidized relative to reduced. Reduction of the CxxC motif in Ost6p causes structural changes only at the peptide-binding groove [30] , confirming that retained peptides bind at this groove rather than through other non-specific interactions [36] . Cell culture growth inhibition assay A total of 4 × 10 3 Human MCF-7 breast tumour cells were cultured in 200 μl of phenol-free media containing 5% charcoal stripped calf serum in 96-well plates. Equal amounts of either human recombinant IFNβ (ProSpec CYT-234), IFN-β WT , IFN-β N101D or no protein were added to the cultures with retinoic acid (Sigma) and incubated for 4 days as described [46] . Cells were fixed with a final concentration of 3.3% (wt/vol) TCA and stained with Sulforhodamine B (Sigma R2625) as described [47] , after which the OD was measured at 490 nm. A control plate to determine initial seeding intensity was included where cells were fixed 2–3 h after plating. Absorbance with this plate was set as 0% growth, and growth obtained with untreated cells was taken as 100%. How to cite this article: Tan, N. Y. et al. Sequence-based protein stabilization in the absence of glycosylation. Nat. Commun. 5:3099 doi: 10.1038/ncomms4099 (2014).